Charge-ordering cascade with spin–orbit Mott dimer states in metallic iridium ditelluride Spin–orbit coupling results in technologically-crucial phenomena underlying magnetic devices like magnetic memories and energy-efficient motors. In heavy element materials, the strength of spin–orbit coupling becomes large to affect the overall electronic nature and induces novel states such as topological insulators and spin–orbit-integrated Mott states. Here we report an unprecedented charge-ordering cascade in IrTe 2 without the loss of metallicity, which involves localized spin–orbit Mott states with diamagnetic Ir 4+ –Ir 4+ dimers. The cascade in cooling, uncompensated in heating, consists of first order-type consecutive transitions from a pure Ir 3+ phase to Ir 3+ –Ir 4+ charge-ordered phases, which originate from Ir 5 d to Te 5 p charge transfer involving anionic polymeric bond breaking. Considering that the system exhibits superconductivity with suppression of the charge order by doping, analogously to cuprates, these results provide a new electronic paradigm of localized charge-ordered states interacting with itinerant electrons through large spin–orbit coupling. Interplay between spin–orbit coupling (SOC) and Coulomb interaction has become a challenging subject in condensed matter physics since it may realize novel superconductivity competing with charge ordering (CO) of spin–orbit Mott states as in the high T C cuprates [1] , [2] , [3] . On the other hand, a charge modulation can be induced by electronic Peierls instability, the so called charge density wave (CDW) [4] , [5] . As electron states are localized as in the Mott states, it appears as a charge order-type modulation due to intersite Coulomb interactions [6] , [7] , [8] . In a system with heavy elements, the large SOC can stabilize the localized spin–orbit Mott state as observed in iridates [9] , and then the charge-ordered Mott state naturally leads a novel electronic framework of the interplay. Further, if the localized Mott state interacts with itinerant conduction electrons, the system possibly experiences valence fluctuations as in the 4 f rare-earth materials [10] and exhibits unprecedented physical phenomena. IrTe 2 was reported as a new CDW material with a modulation vector q =(1/5 0 1/5) below a CDW transition temperature T C ∼ 260 K and also as a mother compound of Ir based superconductors [11] , [12] , [13] . Various efforts have been conducted to elucidate electronic mechanisms of the charge modulation [11] , [13] , [14] , but the CDW like nature was disputable. A recent X-ray diffraction (XRD) study suggested charge modulations not only in the Te site but also in the Ir site with dimerization below T C [15] , suggesting a possibility of the Ir site CO. IrTe 2 is crystallized in a CdI 2 -type layered hexagonal structure ( P3m1 ) with van der Waals bond gap ( Fig. 1a ). The lattice constants at 300 K are a =3.93 Å and c =5.39 Å with c / a =1.37, which is much smaller than c / a =1.6–1.8 in other isostructural dichalcoginides [16] , [17] . The interlayer Te–Te distance (3.50 Å) is also greatly shorter than the expected van der Waals bond length 2 R vdW =4.12 Å, twice of the atomic radius, indicating strong interlayer coupling through the Te–Te covalent bonding. The short bond length is considered as formation of Te 2 3− polymeric bonds [17] . The band calculations predict a three dimension-like Fermi surface with a nesting instability near q =(1/5 0 1/5) and Ir 3+ and Te 1.5− valences in the high temperature (HT) phase [11] . 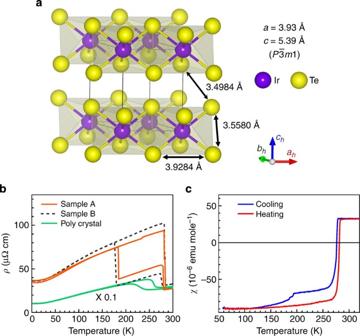Figure 1: Crystal structure and physical properties of IrTe2. On cooling, IrTe2crystals exhibit remarkable thermal hysteretic electrical and magnetic behaviours with consecutive transitions at∼280 and∼180 K but only a single transition at∼280 K on heating, differently from the polycrystalline sample. (a) Each hexagonal layer consists of edge-shared IrTe6octahedrons. The hexagonal axes are presented with red (ah), green (bh) and blue (ch) arrows. Blue and yellow ball symbols are represents Ir and Te atoms, respectively. The interlayer Te–Te bond length (3.4984 Å) is much shorter than the expected van der Waals bond length 2RvdW=4.12 Å. (b) The resistivity results of the single-crystal samples (orange and dotted black lines) display the consecutive transitions accompanied with abrupt changes on cooling, while it does only a single transition on heating. In the resistivity of the polycrystalline sample (green line), which is scaled down to 0.1, the second transition does not appear, indicating that it suppressed by impurities or defects. (c) Magnetic susceptibility is measured with a bunch of IrTe2crystals grown in a single batch to compensate the low magnetic signal. Blue and red lines are measured in cooling and heating, respectively. The susceptibility shows the Pauli paramagnetism above∼280 K but does diamagnetism below∼280 K. On cooling, the susceptibility is further reduced in the second transition, which is not recovered in heating cycle, consistently with the resistivity. Figure 1: Crystal structure and physical properties of IrTe 2 . On cooling, IrTe 2 crystals exhibit remarkable thermal hysteretic electrical and magnetic behaviours with consecutive transitions at ∼ 280 and ∼ 180 K but only a single transition at ∼ 280 K on heating, differently from the polycrystalline sample. ( a ) Each hexagonal layer consists of edge-shared IrTe 6 octahedrons. The hexagonal axes are presented with red ( a h ), green ( b h ) and blue ( c h ) arrows. Blue and yellow ball symbols are represents Ir and Te atoms, respectively. The interlayer Te–Te bond length (3.4984 Å) is much shorter than the expected van der Waals bond length 2 R vdW =4.12 Å. ( b ) The resistivity results of the single-crystal samples (orange and dotted black lines) display the consecutive transitions accompanied with abrupt changes on cooling, while it does only a single transition on heating. In the resistivity of the polycrystalline sample (green line), which is scaled down to 0.1, the second transition does not appear, indicating that it suppressed by impurities or defects. ( c ) Magnetic susceptibility is measured with a bunch of IrTe 2 crystals grown in a single batch to compensate the low magnetic signal. Blue and red lines are measured in cooling and heating, respectively. The susceptibility shows the Pauli paramagnetism above ∼ 280 K but does diamagnetism below ∼ 280 K. On cooling, the susceptibility is further reduced in the second transition, which is not recovered in heating cycle, consistently with the resistivity. Full size image Here we report unprecedented CO behaviours without losing metallicity in a hexagonal layered IrTe 2 . The CO behaviours are investigated by using comprehensive experimental and theoretical studies. The experimental results obtained from a variety of transport and spectroscopic measurements manifest that the system undergoes first order-type consecutive transitions from a pure Ir 3+ to Ir 3+ –Ir 4+ charge-ordered phases with q 1/5 =(1/5 0 1/5) and q 1/8 =(1/8 0 1/8) on cooling while it directly transits from the low temperature (LT) q 1/8 phase to the HT Ir 3+ phase on heating. The transitions involve Ir 5 d to Te 5 p charge transfer with Te anionic polymeric bond breaking. Theoretical free energy model analyses show that the charge-ordered phases are stabilized by localized Ir 5 d spin–orbit Mott states together with diamagnetic Ir 4+ –Ir 4+ dimerization. These results provide a new electronic paradigm of the spin–orbit driven charge-ordered Mott states interacting with itinerant conduction electrons. Electrical and magnetic behaviours The resistivity of high-quality IrTe 2 single crystals exhibits remarkably different behaviours for cooling and heating processes ( Fig. 1b ). On cooling, it shows consecutive resistivity jumps at T C 1 ≈280 K and at T C 2 ≈180 K without losing metallicity. Meanwhile, on heating, the LT phase directly transits into the HT phase at T H ≈280 K with the corresponding resistivity drop. All the transitions are first order-type transitions with ∼ 1 K narrow temperature windows, indicating minimal defects in the crystal. The magnetic susceptibility also displays the uncompensated thermal hysteretic behaviour ( Fig. 1c ). In the HT phase, it shows weak Pauli paramagnetism, which is well explained by the non-magnetic Ir 3+ (5 d 6 ) with the t 2g band full and Te 2 3− with 5 p conduction electrons (one hole per formula unit). On cooling across T C 1 , it drops to be negative and the intermediate phase is diamagnetic. The diamagnetism becomes stronger below T C 2 . In a heating process, it shows the direct LT to HT phase transition at T H as can be seen in the resistivity results. Considering the Ir–Ir dimerization across T C 1 (ref. 15 ), one can suspect the formation of diamagnetic Mott dimer states in analogous to diamagnetic Ti 2 O 3 with dimerized S =1/2 Mott states [18] so that the enhanced diamagnetism reflects increase of the dimer population in the LT phase. Structural identification We performed XRD measurements along a (0 0 4) to (1 0 5) direction ( Fig. 2a,b ) and monitored the ordering peak intensities ( Fig. 2c,d ) at different temperatures. At 300 K, only the Bragg peaks are observable. On cooling ( Fig. 2a,c,e ), the q 1/5 =(1/5 0 1/5) ordering peaks additionally appear at T C 1/5 ≈280 K ( T C 1 ) with a first-order HT to q 1/5 phase transition. The peak intensity maintains nearly constant down to T C 1/8 ≈180 K ( T C 2 ). For further cooling below T C 1/8 , the q 1/5 peaks are suddenly replaced with q 1/8 =(1/8 0 1/8) ordering peaks, and the system undergoes another first order q 1/5 to q 1/8 phase transition. The appearance of the q 1/8 peaks accompanies large increase of a diffusive scattering background, which is due to lack of regularity in the q 1/8 modulation. The peak intensity barely varies with temperature down to 10 K. On heating ( Fig. 2b,d,f ), the q 1/8 peak intensity remains up to T H 1/8 ≈280 K ( T H ) without appearance of the q 1/5 peaks. Meanwhile, the background is somewhat reduced, indicating certain improvement of the q 1/8 regularity. For further heating, the q 1/8 peaks finally disappear across T H 1/8 , and the q 1/8 phase directly transits to the HT phase. One can notice gradual increase of the peak intensity in heating, especially from 200 to 280 K, mainly due to improvement of the modulation regularity. An additional 1/11 ordering of a minor faction was observed in LT phase in the scanning tunnelling microscope (STM) [19] . However, any hint of this order is not observable in the XRD, indicating that it is a surface phenomenon. The q 1/8 regularity degradation may be attributed to smaller domain formation, but can also be considered as a hint of valence fluctuations of the localized Ir 5 d Mott states interacting with the Te 5 p conduction electrons. 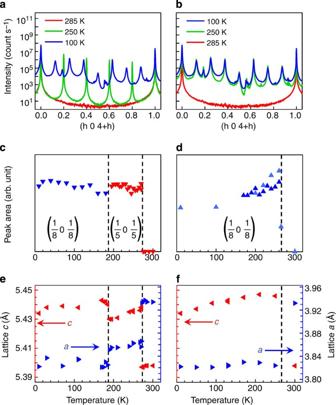Figure 2: Superlattice peaks in IrTe2in cooling and heating processes. XRD data in cooling (a,c,e) and heating (b,d,f) processes. (a) On cooling,q1/5=(1/5 0 1/5) peaks at 250 K (belowTC1/5≈280 K) are replaced with theq1/8=(1/8 0 1/8) peaks at 100 K (belowTC1/8≈180 K). (b) On heating, theq1/8peaks are maintained at 250 K and disappear at 300 K (aboveTH1/8≈280 K). Ordering peak intensities as a function of temperature are displayed. Dashed vertical lines indicate phase boundaries. (c) Theq1/5peaks switch into theq1/8peaks acrossTC1/8on cooling. (d) On heating, theq1/8intensity gradually increases above 200 K mainly due to improvement of the modulation regularity. The in-plane (a) and out-of-plane (c) hexagonal lattice constants are displayed as a function of temperature (e) in cooling and (f) heating processes. Thec/aratio change across the transitions involves partial breaks of Te23−polymeric bonds accompanying Ir average valence changes. Figure 2: Superlattice peaks in IrTe 2 in cooling and heating processes. XRD data in cooling ( a , c , e ) and heating ( b , d , f ) processes. ( a ) On cooling, q 1/5 =(1/5 0 1/5) peaks at 250 K (below T C 1/5 ≈280 K) are replaced with the q 1/8 =(1/8 0 1/8) peaks at 100 K (below T C 1/8 ≈180 K). ( b ) On heating, the q 1/8 peaks are maintained at 250 K and disappear at 300 K (above T H 1/8 ≈280 K). Ordering peak intensities as a function of temperature are displayed. Dashed vertical lines indicate phase boundaries. ( c ) The q 1/5 peaks switch into the q 1/8 peaks across T C 1/8 on cooling. ( d ) On heating, the q 1/8 intensity gradually increases above 200 K mainly due to improvement of the modulation regularity. The in-plane ( a ) and out-of-plane ( c ) hexagonal lattice constants are displayed as a function of temperature ( e ) in cooling and ( f ) heating processes. The c / a ratio change across the transitions involves partial breaks of Te 2 3− polymeric bonds accompanying Ir average valence changes. Full size image Figure 2e,f shows variations of the hexagonal lattice constants determined from the Bragg peaks. On cooling ( Fig. 2e ) across the HT to q 1/5 transition, a (in-plane) decreases while c (out-of-plane) increases, resulting in increase of the c / a ratio from 1.37 to 1.40–1.41. The ratio further increases to 1.42 across the q 1/5 to q 1/8 transition. Meanwhile, on heating ( Fig. 2f ) across T H 1/8 , it is reduced back to 1.37 in the HT phase. Considering that the small c / a ratio in the HT phase involves the Te 2 3− polymeric bonding, the increased ratios in the q 1/5 and q 1/8 phases imply certain degrees of the Te 2 3− bond breaking, which leads the Ir valence change from Ir 3+ ( d 6 ) to Ir 4+ ( d 5 ). SOC assisted electronic transition The Ir valence change is examined by using the Ir 4 f core-level photoemission spectroscopy ( Fig. 3a ). At 300 K (HT phase), the Ir 4 f spectrum displays a simple two-peak feature representing the 4 f 7/2 and 4 f 5/2 core-hole final states. Their binding energies correspond to those of Ir 3+ , confirming the Te 2 3− formation. At 260 K ( q 1/5 phase), each peak splits into double peaks with a 0.41-eV separation, showing that IrTe 2 becomes an Ir 3+ –Ir 4+ mixed valence state. This binding energy ( E B ) shift, the so called chemical shift, is similar to that observed in CuIr 2 S 4 with an Ir 3+ –Ir 4+ CO state [20] , [21] . At 100 K ( q 1/8 phase), the Ir 4+ high binding peak intensity overwhelms the Ir 3+ one. 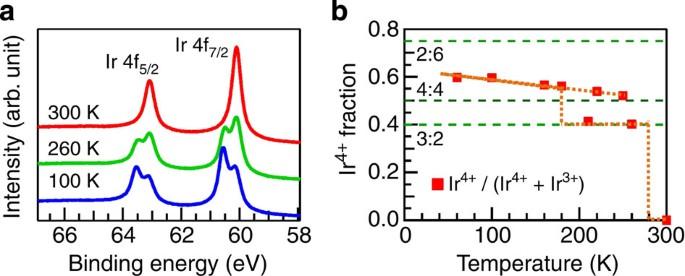Figure 3: Ir valence changes in IrTe2. (a) Ir 4f core-level photoemission spectra at 300 K (HT), 260 K (q1/5) and 100 K (q1/8) are demonstrating Ir valence changes. Single peaks at 300 K indicate pure Ir3+, while mixed Ir3+–Ir4+at 260 and 100 K is evident in high binding peaks (that is, high valence state). (b) Ir4+fractions obtained from the Ir 4f core-level spectra are displayed as a function of temperature. The fraction stays at 2/5 (Ir3+:Ir4+=3:2) in theq1/5phase, while it varies in a range from 0.5 to 0.6 in theq1/8phase. The green lines indicate characteristic ratio ofq1/5(3:2), (3212)-typeq1/8(4:4) and (12212)-typeq1/8(2:6) orderings. Figure 3b shows the Ir 4+ fractions for different temperatures and phases estimated from the Ir 3+ and Ir 4+ relative peak intensities ( Supplementary Fig. 1 ). The transitions accompany the Ir average valence changes from a pure Ir 3+ in the HT phase to an Ir 3+ –Ir 4+ mixed valence with a 3:2 fixed ratio in the q 1/5 phase. In the q 1/8 phase, the ratio becomes (4− x ):(4+ x ) with monotonic increase of the x -value from zero near T H 1/8 to about one below 50 K, indicating the Ir 5 d valence fluctuation. The appearance of Ir 4+ , which reflects the Te 2 3− polymeric bond break to yield Te 2− , verifies that the q 1/5 and q 1/8 modulations involve Ir 3+ –Ir 4+ charge orders. Figure 3: Ir valence changes in IrTe 2 . ( a ) Ir 4f core-level photoemission spectra at 300 K (HT), 260 K ( q 1/5 ) and 100 K ( q 1/8 ) are demonstrating Ir valence changes. Single peaks at 300 K indicate pure Ir 3+ , while mixed Ir 3+ –Ir 4+ at 260 and 100 K is evident in high binding peaks (that is, high valence state). ( b ) Ir 4+ fractions obtained from the Ir 4f core-level spectra are displayed as a function of temperature. The fraction stays at 2/5 (Ir 3+ :Ir 4+ =3:2) in the q 1/5 phase, while it varies in a range from 0.5 to 0.6 in the q 1/8 phase. The green lines indicate characteristic ratio of q 1/5 (3:2), (3212)-type q 1/8 (4:4) and (12212)-type q 1/8 (2:6) orderings. 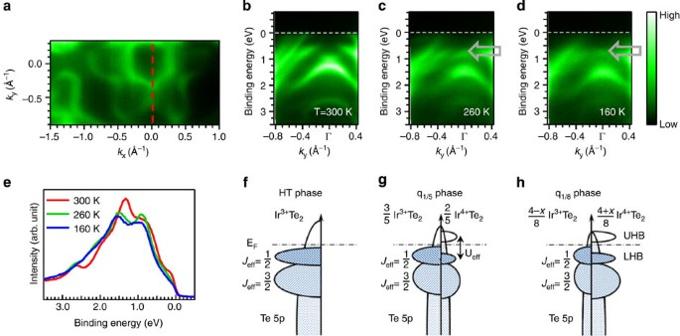Figure 4: Electronic structure of IrTe2. (a) Fermi surface topology in the Γ-sheet (kz=5c*) obtained from ARPES at 300 K. It displays a sixfold flower shape as predicted in a band calculation. (b–d) Angle-resolved spectra for the Γ-cut (red dotted line ona) at different temperatures. At 300 K (HT phase), the spectra are much coherent because the system has no CO. An additional flat band atEB∼0.8 eV, which represents the spin–orbit low Hubbard band (LHB), appears around the Γ-point at 260 K and is extended at 160 K in the k-space. The spectra belowTC1/5(260 K) become less coherent because of an alternating potential difference of Ir3+and Ir4+as well as the monoclinic distortion. Further broadening at 160 K is attributed to the irregular domain formation ofq1/8charge order. (e) Angle-integrated spectra are displayed. The spectral weight atEFdecreases belowTC1/5and does more belowTC1/8(f–h) Schematic energy diagrams in the three different phases. At HT phase (f), the spin–orbit coupled Jeff=3/2 and Jeff=1/2 bands are fully occupied by six electrons at Ir3+(5d6) sites, while the Te 5pband crossesEFwith one hole per formula unit. Atq1/5phase (g), the hole transfers into the Ir 5dand Ir4+(5d5) forms the spin–orbit Mott state with the upper and lower Hubbard bands (UHB and LHB) separated byUeff, which is enhanced by the dimer formation. Atq1/8phase (h), the population of Ir4+dimer increases and the valence fluctuation is exhibited as a function of temperature. Full size image Figure 4a–d show the Fermi surface topology around the Γ-point at 300 K obtained by using the angle-resolved photoemission spectroscopy (ARPES) and the Γ-cross ARPES spectra in three different phases, respectively. The predicted electronic structure well agrees with the ARPES results in the HT phase ( Supplementary Fig. 2 ). The transitions accompany considerable spectral changes not only at the Fermi level ( E F ) but also in the 0–3 eV valence band region. The spectral weight at E F gradually decreases with cooling from 300 to 260 K and to 100 K without losing the metallic E F feature as shown in Fig. 4e , consistently with the optical results across the HT to q 1/5 phase transition [14] . These results well explains the resistivity jumps across the transitions (see Fig. 1b ). The electronic changes across the transitions are also observable in the Γ-cross band dispersions ( Fig. 4b–d ). The overall dispersions are mostly maintained across the transitions. However, one can notice that an additional flat band feature appears at E B ∼ 0.8 eV in the q 1/5 phase and is extended in the q 1/8 phase. Figure 4: Electronic structure of IrTe 2 . ( a ) Fermi surface topology in the Γ-sheet ( k z =5 c *) obtained from ARPES at 300 K. It displays a sixfold flower shape as predicted in a band calculation. ( b – d ) Angle-resolved spectra for the Γ-cut (red dotted line on a ) at different temperatures. At 300 K (HT phase), the spectra are much coherent because the system has no CO. An additional flat band at E B ∼ 0.8 eV, which represents the spin–orbit low Hubbard band (LHB), appears around the Γ-point at 260 K and is extended at 160 K in the k-space. The spectra below T C 1/5 (260 K) become less coherent because of an alternating potential difference of Ir 3+ and Ir 4+ as well as the monoclinic distortion. Further broadening at 160 K is attributed to the irregular domain formation of q 1/8 charge order. ( e ) Angle-integrated spectra are displayed. The spectral weight at E F decreases below T C 1/5 and does more below T C 1/8 ( f – h ) Schematic energy diagrams in the three different phases. At HT phase ( f ), the spin–orbit coupled J eff =3/2 and J eff =1/2 bands are fully occupied by six electrons at Ir 3+ (5 d 6 ) sites, while the Te 5 p band crosses E F with one hole per formula unit. At q 1/5 phase ( g ), the hole transfers into the Ir 5 d and Ir 4+ (5 d 5 ) forms the spin–orbit Mott state with the upper and lower Hubbard bands (UHB and LHB) separated by U eff , which is enhanced by the dimer formation. At q 1/8 phase ( h ), the population of Ir 4+ dimer increases and the valence fluctuation is exhibited as a function of temperature. Full size image The electronic structures in the three different phases can be described schematically in Fig. 4f–h . The Ir 5 d state is split into a triplet t 2g and a doublet e g states with a splitting energy 10 Dq ∼ 3 eV under the octahedral O h symmetry. The large SOC energy ( ∼ 0.5 eV) of Ir 5 d splits again the low lying t 2g states into the spin–orbit J eff =3/2 and J eff =1/2 states [9] . In the HT phase with pure Ir 3+ (5 d 6 ), both the J eff =3/2 and J eff =1/2 bands are fully occupied while the Te 5 p wide band crosses E F with one hole per Te 2 3− . On cooling across T C 1/5 ( q 1/5 phase), the Te 2 3− bonds are partially broken with Ir 5 d to Te 5 p electron transfer, and the system becomes a 3:2 Ir 3+ –Ir 4+ charge-ordered state. At the Ir 4+ (5 d 5 ) site, the J eff =1/2 state becomes half-full, and the electronic state is expected to become the localized J eff =1/2 Mott state as in Sr 2 IrO 4 . The dimerization leads the diamagnetic spin–orbit Mott dimer states, and the Hubbard U , which is <1 eV in Sr 2 IrO 4 , is effectively enlarged by the dimerization energy (Δ) to be U eff (= U +Δ) ∼ 1.5 eV. The newly appearing flat band at E B ∼ 0.8 eV seems to represent the low Hubbard band of the spin–orbit Mott dimer state. The characteristic orbital occupation ratio n xy : n yz : n zx =1:1:1 for the t 2g xy , yz and zx orbitals in the J eff =1/2 state [4] should be adjusted by the dimerization, which relatively lowers the energy of xy orbital along the dimer direction. A molecular field calculation for an Ir 4+ –Ir 4+ dimer shows that the occupation ratio becomes roughly n xy : n yz : n zx =2:1:1 for Δ ∼ 0.7–0.8 eV, as predicted in the band calculations for the q 1/5 phase [15] . The Ir 5 d to Te 5 p charge transfer reduces the density of state at E F to drive the resistivity jump. In the q 1/8 phase, the Ir 4+ fraction increases and the carrier density further decreases. Real space ordering patterns and phase diagrams The real space ordering patterns are investigated by using the STM measurements from a cleaved (001) surface as shown in Fig. 5 . The stripe type modulations are clearly observable along the [100] direction in the ordered phases. The layered structure naturally yields the Te layer at the surface, and the STM image reflects the tunnelling current through the Te 5 p states, which is determined by the local charge carrier density and relative vertical heights of Te ions on the surface. The CO occurs at the Ir sites and the Te 5 p local charge density and vertical height are affected by the neighbouring Ir states. Thus, the observed modulation in the Te layer reflects the Ir 3+ –Ir 4+ charge order in the underneath Ir layer. The STM image in the q 1/5 phase ( Fig. 4a ) is well explained by the Te 5 p charge modulation formed by a (32)-type [Ir 3+ Ir 3+ Ir 3+ ][Ir 4+ Ir 4+ ] q 1/5 charge order. This pattern represents the two-dimensional charge order in the Ir layer projected from the q 1/5 =(1/5 0 1/5) three-dimensional order ( Supplementary Fig. 3 ), and well matches with the Ir arrays determined from the XRD analyses [15] ( Supplementary Fig. 4 ). In the q 1/8 phase, two types of the 1/8 modulations are observable and understood with the modulations by a (3212)-type [Ir 3+ Ir 3+ Ir 3+ ][Ir 4+ Ir 4+ ][Ir 3+ ][Ir 4+ Ir 4+ ] order with 4Ir 3+ :4Ir 4+ ( Fig. 5b ) and a (12212)-type [Ir 3+ ][Ir 4+ Ir 4+ ][Ir 4+ Ir 4+ ][Ir 3+ ][Ir 4+ Ir 4+ ] with 2Ir 3+ :6Ir 4+ ( Fig. 5c ). The (3212)-type is dominant but the (12212)-type fraction increases on cooling to yield Ir 3+ :Ir 4+ =(4− x ):(4+ x ) with increasing x as observed in the Ir 4 f core-level study (see Fig. 3b ). The Ir 5 d valence fluctuation admixes the two q 1/8 order types and likely degrades the modulation regularity to enhance the scattering background (see Fig. 2a ). 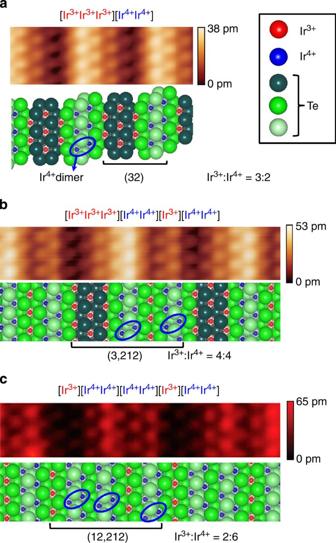Figure 5: STM images with atomic arrangements. STM images of each phase are displayed with atomic arrangement. Red and blue spheres represents Ir3+and Ir4+ion, respectively. Two neighbouring Te ions get closer to each other due to the underneath Ir4+–Ir4+dimer (blue ellipse). The lattice distortion changes the height of Te ions, which locates between two dimerized Ir4+ions and results bright signal on STM image. (a) STM image in theq1/5phase is compared with the atomic arrangements for the (32)-typeq1/5order. (b,c) STM images in (3212)-typeq1/8phase and (12212)-type q1/8 phase are displayed with relevant atomic arrangement. The Ir4+ions always appear in pair (diamagnetic dimer formation). Figure 5: STM images with atomic arrangements. STM images of each phase are displayed with atomic arrangement. Red and blue spheres represents Ir 3+ and Ir 4+ ion, respectively. Two neighbouring Te ions get closer to each other due to the underneath Ir 4+ –Ir 4+ dimer (blue ellipse). The lattice distortion changes the height of Te ions, which locates between two dimerized Ir 4+ ions and results bright signal on STM image. ( a ) STM image in the q 1/5 phase is compared with the atomic arrangements for the (32)-type q 1/5 order. ( b , c ) STM images in (3212)-type q 1/8 phase and (12212)-type q1/8 phase are displayed with relevant atomic arrangement. The Ir 4+ ions always appear in pair (diamagnetic dimer formation). Full size image Now we compare free energies, F = E − TS , for the charge configuration states of the uniform Ir 3+ (HT), and the Ir 3+ –Ir 4+ -ordered states with the q 1/5 (32)-type, q 1/8 (3212)-type and q 1/8 (12212)-type ( Supplementary Table 1 , Supplementary Note 1 ). Within a mean-field description, the energy E for each state with the spin–orbit Mott dimer states can be simply expressed in terms of the Te 5 p (Ir 5 d ) hole energy ɛ p(d) , the Ir 4+ –Ir 4+ dimerization energy Δ, the nearest neighbor intersite d – d Coulomb energy V dd , the p – d valence sharing energy U pd and the lattice energy ɛ L (see equation (1) in Methods). The entropy changes across the transitions are estimated from the specific heat measurements ( Supplementary Fig. 5 ). In spite of simplicity, the free energy analysis, in which V dd and Δ play critical roles to drive the CO, can successfully reproduce the transitions observed in IrTe 2 . The resulting phase diagrams are presented for cooling ( Fig. 6a ) and heating ( Fig. 6b ) processes. On cooling, the system undergoes consecutive transitions at k B T C 1/5 / V dd =0.100 (HT to q 1/5 ) and at k B T C 1/8 / V dd =0.063 ( q 1/5 to q 1/8 ) for (Δ/2+ ɛ p − ɛ d )/ V dd =0.98, yielding T C 1/5 =278 K and T C 1/8 =175 K for V dd =0.24 eV in a good agreement with the observed T C 1/5 ∼ 280 K and T C 1/8 ∼ 180 K. In the heating process, we additionally introduced a small q 1/8 pinning energy of 0.0013 V dd (0.31 meV) per formula unit, which completely suppresses the q 1/5 phase and leads to the direct q 1/8 to HT phase transition at T H 1/8 =282 K, 4 K higher than T C 1/5 as observed in the resistivity and specific heat data (see Fig. 1b and Supplementary Fig. 5 ). In the q 1/8 phase, the free energies of the (12212)- and (3212)-type ordered states are close to each other, reflecting their coexistence. Suppose the Ir 5 d to Te 5 p charge transfer energy ɛ d − ɛ p ∼ 0.1 eV, which corresponds to the Ir 5 d binding energy at the Ir 3+ site ( d 6 → d 5 ), the dimerization energy Δ is ∼ 0.7 eV with V dd =0.24 eV. 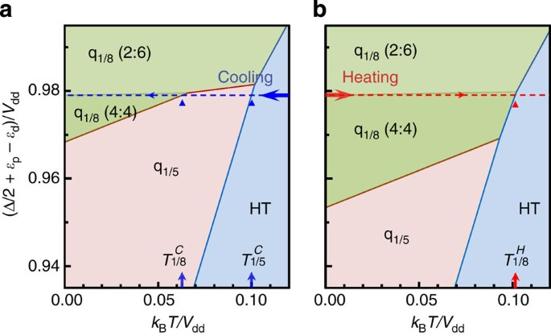Figure 6: Phase diagrams of IrTe2. Phase diagrams obtained from free energy analyses for (a) cooling and (b) heating. Model parameters—Te 5p energy (ɛp), Ir 5d energy (ɛd), dimer formation energy (Δ) and temperature (T)—are renormalized with an intersite Coulomb interaction (Vdd). Blue and pink regions denote the non-ordered HT andq1/5ordered phases, respectively. Light and dark green regions representq1/8(4:4) andq1/8(2:6) ordered phases with the (3212)- and (12212)-type charge orders, respectively. Figure 6: Phase diagrams of IrTe 2 . Phase diagrams obtained from free energy analyses for ( a ) cooling and ( b ) heating. Model parameters—Te 5p energy ( ɛ p ), Ir 5d energy ( ɛ d ), dimer formation energy (Δ) and temperature ( T )—are renormalized with an intersite Coulomb interaction ( V dd ). Blue and pink regions denote the non-ordered HT and q 1/5 ordered phases, respectively. Light and dark green regions represent q 1/8 (4:4) and q 1/8 (2:6) ordered phases with the (3212)- and (12212)-type charge orders, respectively. Full size image IrTe 2 exhibits unprecedented physical properties with various unusual features such as the uncompensated thermal hysteretic transition behaviour, multiple charge-ordered states without losing metallicity, anionic polymeric bond breaking, dimerization and charge fluctuation. It is noticed that the q 1/5 to q 1/8 phase transition is a commensurate to commensurate first-order transition and can be considered as a rare ‘harmless’ stair case [22] , distinguishable from the commonly observed devil’s stair case [23] . The commensurate q 1/8 phase seems to be pinned by the lattice, and directly transits into the HT phase without appearance of the q 1/5 phase on heating. The unique behaviour in IrTe 2 is driven by the localized spin–orbit Mott dimer states. The results offer a novel electronic paradigm, in which localized charge-ordered states interact with conduction electrons introduced by the large SOC and the interplay between SOC and Coulomb interaction plays essential roles. Pd or Pt doping, introducing additional electrons, suppresses the charge order and the system becomes a superconductor at LT [11] , [12] , [13] . It indicates that the superconducting order competes with the charge order, similarly as in the cuprates [1] , [2] , [3] although the mechanism can be different, and suggests a possibility for realization of superconductivity involving the spin–orbit Mott state. Single-crystal preparation and transport measurements High-quality IrTe 2 single crystals were grown by using a chemical vapour transport method from the Te flux. The electrical resistivity and magnetic susceptibility were measured by using commercial physical property measurement system and magnetic property measurement system, respectively. The second transition temperature T C 2 is sensitive to the sample quality and varies in a range from 185 to 170 K among the crystals even from a single batch. The second transition is even not observable in the crystals prepared through fast cooling from the growth temperature. We obtained the magnetic signal from a bunch of single crystals (13 mg) grown in a single batch to improve the signal to noise ratio so that it displays a multi-domain behaviour for the second transition in the magnetic susceptibility. XRD measurements The superstructure in IrTe 2 was investigated by using hard XRD measurement at the 3A beamline in Pohang Light Source with six-circle PSI diffractometer. The photon energy was set to be 10.8 keV ( λ =1.148 Å), a pre-edge of Ir L 3 white line (11.2 keV). The temperature was controlled within ±0.5 K. The diffracted photon flux were monitored through a scintillator (NaI:Tl). The order parameters were estimated from the (1/5 0 4+1/5) and (1/8 0 4+1/8) ordering peak intensities in the q 1/5 and q 1/8 phases, respectively. ARPES and STM measurements For ARPES and STM measurements, the single crystals were cleaved in situ at 300 K in a ultrahigh vacuum better than 8 × 10 −11 Torr by using a post method to expose a clean (001) surface with the Te layer termination. ARPES was performed at the 4A1 beamline in Pohang Light Source with a Scienta SES-2002 electron spectrometer. We used linearly polarized light in the photoelectron scattering plane. The inner potential was found to be V 0 =13 eV for the crystal momentum (Å −1 ) along the crystal c -axis, which yields E kin =116.89 eV at Γ(≈5c*) point and E kin =92.33 eV at A point (≈4.5c*) for the lattice parameter c =5.386 Å. The total energy resolution was set to be ∼ 85 meV. The STM images were obtained in a constant-current mode with the tunnelling current of ∼ 0.1 nA. The atomic arrays are drawn by using VESTA software [24] . Free energy model analysis Considering the ordered structures, in which each (1 0 1) plane consists of IrTe 6 octahedrons with purely either Ir 3+ or Ir 4+ , the system is effectively reduced to a one-dimension (1D) chain along the [1 0 1] direction. Suppose that the system is a 1D chain with N -unit (IrTe 2 ) cell lattice sites, the energy per unit cell is expressed within a mean-field description as where n p(d) denote the average number of the Te 5 p (Ir 5 d ) holes. The d hole number at the i -site is set to be for Ir 3+ and for Ir 4+ , and the total number of holes is constrained to be one, that is, n p + n d =1. How to cite this article: Ko, K.-T. et al . Charge-ordering cascade with spin–orbit Mott dimer states in metallic iridium ditelluride. Nat. Commun. 6:7342 doi: 10.1038/ncomms8342 (2015).